Oceanic spawning ecology of freshwater eels in the western North Pacific The natural reproductive ecology of freshwater eels remained a mystery even after some of their offshore spawning areas were discovered approximately 100 years ago. In this study, we investigate the spawning ecology of freshwater eels for the first time using collections of eggs, larvae and spawning-condition adults of two species in their shared spawning area in the Pacific. Ovaries of female Japanese eel and giant mottled eel adults were polycyclic, suggesting that freshwater eels can spawn more than once during a spawning season. The first collection of Japanese eel eggs near the West Mariana Ridge where adults and newly hatched larvae were also caught shows that spawning occurs during new moon periods throughout the spawning season. The depths where adults and newly hatched larvae were captured indicate that spawning occurs in shallower layers of 150–200 m and not at great depths. This type of spawning may reduce predation and facilitate reproductive success. The reproductive ecology of anguillid eels far offshore in the oceans has remained enigmatic even though it has been known that they must aggregate and spawn within estimated spawning areas. These spawning areas have been historically located by catching their small leaf-like larvae called leptocephali, first in the Sargasso Sea of the North Atlantic [1] and then more recently in the western North Pacific [2] . Spawning in the western North Pacific was recently corroborated by catching adult eels [3] , but no eggs were collected in these spawning areas [4] . Their long migrations to these spawning areas have fascinated scientists because each eel must swim thousands of kilometres back to the same area where it was born and then find a mate to spawn with [4] . Migrating eels of a few species have been caught incidentally along continental margins in both the Atlantic and Pacific oceans, but never close to their spawning areas [4] , [5] . Information has been obtained about their migration behaviour using high-technology satellite tags, which have shown that migrating eels usually swim at deeper depths of about 500–900 m during the day and at shallower depths of 100–300 m at night [6] , [7] . Swimming at such deep daytime depths during migration may be related to predator avoidance, or to regulating the maturation process using different water temperatures [6] , [7] , [8] . However, none of these tagging studies have documented the behaviour of eels that clearly reached their spawning areas. Until recently [3] , various published and unpublished attempts in the last 30 years to capture or observe adult eels within their spawning areas have failed in both the Sargasso Sea [9] and western North Pacific [10] . Success in artificially inducing maturation of eels have enabled some spawning behaviour to be observed in the laboratory [11] , [12] and their cultured leptocephali have been studied in recent years [13] , [14] . The laboratory observations of spawning adults have suggested the possibility of group spawning by anguillid eels [11] , [12] , but these observations provide limited understanding of the natural reproductive ecology of eels. Questions about the biological characteristics of spawning eels, when and how deep they spawn in the ocean, or how they find each other and form spawning aggregations, have remained unanswered because of the inability to catch or observe adult eels in their spawning areas. In the western North Pacific, the spawning area of the Japanese eel, Anguilla japonica , was found to be located in the westward flowing North Equatorial Current to the west of Guam, by catching their small larvae [2] . Catches of all sizes of larvae of the tropical species the giant mottled eel, Anguilla marmorata , together with the larvae of the temperate species the Japanese eel, have also indicated that both species use the same spawning area in the North Equatorial Current [15] , even though their larvae eventually recruit to different regions ranging from Japan to Indonesia. To facilitate conservation efforts for these eels, and for freshwater eels in general, which are increasingly endangered globally [16] , [17] , the spawning area in the western North Pacific has been intensively studied recently. In this study, we aimed to understand the reproductive ecology of freshwater eels using larval sampling surveys from 2005 to 2009 and trawling surveys in 2008 and 2009 to capture adult eels in this estimated spawning area. Large midwater trawls were used to collect adult eels, and large plankton nets were used to collect their eggs and larvae, in conjunction with hydrographic surveys of the structure of the ocean. DNA sequences were used to identify the species of the collected specimens and various morphological or physiological observations were made on the captured adults. The spatial and temporal patterns of these catches of adults, eggs and larvae showed that both species appeared to be spawning in the upper few hundred metres of the ocean during new moon periods to the west of the seamount chain, and the reproductive characteristics of the adults indicated that they might be able to spawn more than once during the spawning season. We suggest that shallow spawning on dark new moon nights near the seamount chain likely facilitates synchronization of spawning aggregations and reduces predation on adults and eggs. Catches of adult eels During the adult eel surveys, a total of 62 horizontal tows of large 900–3,000 m 2 mouth opening scientific trawls were made mostly at night at depths of 132–766 m from June to August of 2008 and from May to June of 2009. 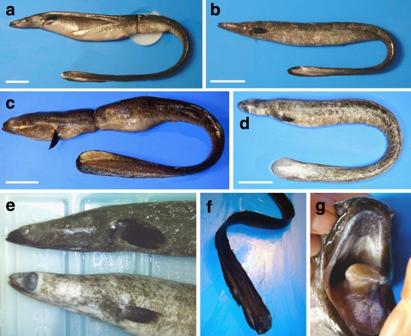Figure 1: Spawning-condition adult freshwater eels. (a) Female Japanese eel,Anguilla japonica, 749 mm in length with unfertilized eggs that flowed out of the genital pore after collection (dish in photo). Scale bar, 50 mm. (b) MaleA. japonica(447 mm). Scale bar, 50 mm. (c) Female giant mottled eelAnguilla marmorata(1,223 mm). Scale bar, 100 mm. (d) MaleA. marmorata(457 mm). Scale bar, 50 mm. (e) Comparison of the anterior part of the bodies of maleA. japonica(top: 585 mm) and theA. marmoratain (d) (bottom) that were caught together in the same net, showing a greater enlargement of the eyes inA. marmoratathan inA. japonica. (f) Tail part of a maleA. japonica(471 mm) that was still in good condition for swimming despite its very thin body. (g) Degenerated teeth of the upper jaw of the femaleA. marmoratain (c). Nine of these tows deployed at 163–303 m depth layers caught a total of 15 adult freshwater eels ( Table 1 , Fig. 1 ). A. japonica (six males and six females, Fig. 1a,b,e,f ) and giant mottled eels (two males and one female, Fig. 1c–e,g ) were collected at three different latitudes along the southern part of the West Mariana Ridge seamount chain ( Fig. 2 ) in June [3] and August 2008 (ref. 18 ), and in June 2009. These eels were caught around new moon periods of each month (4 days before to 2 days after the new moon, Fig. 3a ) despite considerable sampling effort before (−10 days) and after (+6 days) the new moon ( Supplementary Table S1 ). The timing of these collections of adults also overlapped with the collections of eggs and recently hatched preleptocephali (prefeeding-stage larvae; Fig. 3b,c ). Table 1 Catches and biological characteristics of two species of adult freshwater eels. Full size table Figure 1: Spawning-condition adult freshwater eels. ( a ) Female Japanese eel, Anguilla japonica , 749 mm in length with unfertilized eggs that flowed out of the genital pore after collection (dish in photo). Scale bar, 50 mm. ( b ) Male A. japonica (447 mm). Scale bar, 50 mm. ( c ) Female giant mottled eel Anguilla marmorata (1,223 mm). Scale bar, 100 mm. ( d ) Male A. marmorata (457 mm). Scale bar, 50 mm. ( e ) Comparison of the anterior part of the bodies of male A. japonica (top: 585 mm) and the A. marmorata in ( d ) (bottom) that were caught together in the same net, showing a greater enlargement of the eyes in A. marmorata than in A. japonica . ( f ) Tail part of a male A. japonica (471 mm) that was still in good condition for swimming despite its very thin body. ( g ) Degenerated teeth of the upper jaw of the female A. marmorata in ( c ). 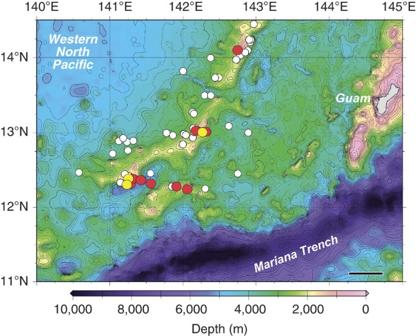Figure 2: Locations where adult eels were collected within their spawning area. Adults of the Japanese eel,Anguilla japonica, are shown with red circles, those of the giant mottled eel,Anguilla marmorata, with yellow circles and tows that collected no adult eels with white circles. Eels were collected in June and August 2008, and in June 2009. Every tow of a trawl is represented with a circle plotted at the midpoint of each deployment. Black scale bar, 50 km. Full size image Figure 2: Locations where adult eels were collected within their spawning area. Adults of the Japanese eel, Anguilla japonica , are shown with red circles, those of the giant mottled eel, Anguilla marmorata , with yellow circles and tows that collected no adult eels with white circles. Eels were collected in June and August 2008, and in June 2009. Every tow of a trawl is represented with a circle plotted at the midpoint of each deployment. Black scale bar, 50 km. 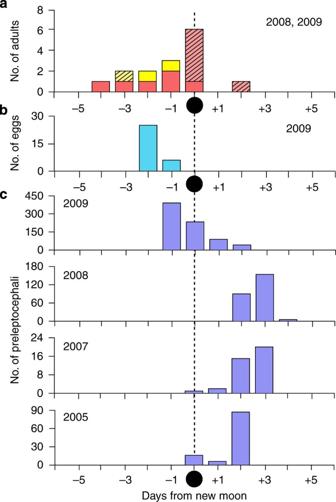Figure 3: Timing of catches of each life history stage in relation to the new moon. (a) Catches of adult eels in June and August 2008, and June 2009 (n=15). Red bars show Japanese eels,Anguilla japonica, and yellow bars the giant mottled eels,Anguilla marmorata, with hatched bars indicating females and solid bars indicating males. (b) Eggs collected in May 2009 (n=31). (c)A. japonicapreleptocephali collected in 2009 (May,n=753), 2008 (June,n=249), 2007 (August,n=38) and 2005 (May,n=110) from top to bottom. All catches are plotted in relation to the date of the new moon of each month, except for twoA. japonicapreleptocephali from a different survey in July 2008 collected at +5 and +7 days, and 31A. marmoratapreleptocephali collected between −3 and +5 days from the new moon in July and August of 2006, and August of 2007. Full size image Figure 3: Timing of catches of each life history stage in relation to the new moon. ( a ) Catches of adult eels in June and August 2008, and June 2009 ( n =15). Red bars show Japanese eels, Anguilla japonica , and yellow bars the giant mottled eels, Anguilla marmorata , with hatched bars indicating females and solid bars indicating males. ( b ) Eggs collected in May 2009 ( n =31). ( c ) A. japonica preleptocephali collected in 2009 (May, n =753), 2008 (June, n =249), 2007 (August, n =38) and 2005 (May, n =110) from top to bottom. All catches are plotted in relation to the date of the new moon of each month, except for two A. japonica preleptocephali from a different survey in July 2008 collected at +5 and +7 days, and 31 A. marmorata preleptocephali collected between −3 and +5 days from the new moon in July and August of 2006, and August of 2007. Full size image Each of the three A. marmorata (two males and one female) was caught with a male A. japonica in the same tows, whereas other multiple catches included only female A. japonica (two and three females). All males were caught in the cod end of trawls and were less damaged, whereas all but one of the females ( A. japonica ) were caught by being entangled in the large-diameter mesh of the side net, which scarred or squeezed their bodies ( Fig. 1a,c ). This may suggest that anguillids form single-sex aggregations before and after spawning, or that the two sexes have different swimming behaviour to avoid capture inside the trawl, but more detailed observations are needed. Examinations of the morphology of these adult eels provided the first information about the condition of spawning anguillids ( Fig. 1 ). All eels were silvery black in colour (especially A. japonica ) with greatly enlarged eyes (especially A. marmorata , Fig. 1e ) and had degenerated teeth due to decalcification ( Fig. 1g ). Body colour of the A. marmorata male in Figure 1d,e was metallic grey, but had many scratches caused by netting. Their bodies were quite thin except in the abdomen area, but they had well-developed caudal and pectoral fins for swimming ( Fig. 1f ). All the eels had significantly degenerated digestive tracts with no visible stomach/intestine contents or evidence of feeding. In addition, the very similar stable isotopic profiles between these eels and the silver eels just starting their spawning migration from East Asia were distinct from those of mesopelagic fishes caught in the spawning area [19] . This suggests that Japanese eels did not assimilate nutrition from the marine environment during their long spawning migration ( ∼ 6 months) and that they retained their initial isotopic values from before migration [19] . Some of the eels caught after spawning were very thin and weak, such as the two females caught in August 2008 (ref. 18 ) that only weighed 91 and 117 g ( Table 1 ), which verified that all these eels die after spawning, as salmon do after they spawn in rivers. A. japonica females were significantly larger in length (mean±s.d. : 674±93 mm, range 555–767 mm) than males (524±74 mm, 447–639 mm; P =0.025), but not in body weight (218±130 g, 91–406 g for females, 144±44 g, 84–200 g for males; P >0.05; Table 1 ). These lengths were similar to those of the migrating eels of this species caught in several areas of coastal Japan that had mean lengths of 661±88–748±90 mm for females and 475±44–590±112 mm for males [20] , [21] . However, the spawning-condition eels were much lighter in weight, as the females from coastal Japan had mean weights of 445±196–739±229 g and males were 144±41–239±74 g (refs 20 , 21 ). The female A. marmorata (1,223 mm, 2,496 g) was also larger than the males of that species (457 and 623 mm, 190 and 314 g). The mean ages of the spawning-condition A. japonica that were estimated by otolith annual rings were 7.0 (females, range 5–10, n =4) and 6.8 (males, range 5–10, n =4) years, and these are similar to the ages of silver eels collected as they leave coastal Japan [20] . The ages of A. marmorata collected in the spawning area were 12 (female, n =1) and 6 (male, N =1) years. Although it is well known that male eels are smaller and younger than females when they start migrating offshore, these data confirmed that the males caught in the spawning area were also smaller and younger than females, and showed that even small males (<450 mm) can succeed in reaching the spawning area. Preliminary microchemical analyses of otolith strontium:calcium (Sr:Ca) ratios of two females and two males of the spawning condition A. japonica showed that one male had lived in a river, two (one male and one female) had inhabited a brackish water estuary and one female had lived in coastal marine habitats during their yellow eel growth phase in continental waters of East Asia. This could be inferred because the Sr concentration is much higher in seawater than in freshwater, and the Sr concentration in the water in which each eel lived was recorded in its otoliths [22] . These eels with various habitat use histories that were collected in the spawing area were similar to eels caught in Japanese coastal waters that were found to have lived in both freshwater and saline habitats [23] . This suggests the importance of conservation of all habitats from freshwater to the estuary and coastal waters for anguillid eels. Reproductive characteristics of eels All females of both species collected in June 2009 had gonads in a post-spawning condition with degenerated follicles after ovulation ( Supplementary Fig. S1 ). However, they showed relatively high gonad-somatic index values of 9.0–13.4% (GSI: relative weight of gonad to body weight; Table 1 ) compared with those of migrating female Japanese eels (only about 1–4% (refs 5 , 20 , 21 , 24 )) just leaving East Asian coastal waters, whereas GSI values of artificially matured eels can reach 40–70% at their spawning [4] . The 739-mm post-spawning condition female A. japonica in Supplementary Figure S1a showed a moderately higher GSI value of 11.2%, compared with migrating eels leaving coastal waters; however, part of this high GSI value is likely due to a loss of body weight and fat reserves that are converted into gonads or energy for locomotion during migration. It had a large, healthy bright red liver and an apparently functioning swim bladder, but the digestive tract was degenerated ( Supplementary Fig. S1a ). Approximately 90% of oocytes in the spawning-condition eel ovaries were at the mid-vitellogenic stage with oocyte diameters of 350–600 μm, whereas those of eels migrating out of coastal waters were at the pre- to early-vitellogenic stages with egg diameters of ∼ 150–300 μm (ref. 24 ). The thickness of the chorion of oocytes in the female A. japonica collected in the spawning area (mean±s.d. : 4.4±0.9 μm, range: 3.2–6.3 μm, n =28) was slightly, but significantly, thinner than those of artificially matured eels (5.1±0.6 μm, 4.0–6.6 μm, n =35) that were induced into vitellogenic growth at the mid- to late-vitellogenic stages ( P <0.05). The relatively advanced maturation stages and larger sizes of the remaining oocytes in the post-spawning females suggested that their ovaries were polycyclic, similar to those of many marine eel species [25] , and that they had the potential to spawn repeatedly 1 or 2 months after the first spawning of the primary egg batch. One female A. japonica caught on 23 June 2009, the day of the new moon (749 mm, 244 g, Eel No.12, Table 1 ), had over-ripened ovulated eggs (mean egg diameter±s.d., 904±117 μm, n =117) in the abdomen, and had 162 g of eggs flow out from its genital pore after collection ( Fig. 1a ). Including all ovulated eggs, its GSI would have been 47.8% ( Table 1 ), whereas the value excluding ovulated eggs was 13.1%. This specimen appeared not to have spawned normally in the last spawning event during the new moon period when it was caught, on the basis of the degenerated characteristics of the eggs, such as the overconflated oil droplets and the fragmentation of the electrophoresis profiles of the RNA extracted from the eggs. In contrast, two other females collected in the late spawning season at the end of August 2008 appeared to be very exhausted and had vestigial ovaries with only a few regressed oocytes [18] , indicating that they had spawned out almost all of their eggs. Although males migrating out of East Asia have GSI values <1% (refs 20 , 21 ), all males of both species collected in the spawning area had well-developed testis with GSI values of 13.4–40.3% ( Table 1 ). One male A. japonica (447 mm, 129 g) collected on 22 June 2009 ( Fig. 1b ) had well-developed testes ( Supplementary Fig. S1b ), with the highest male GSI of 40.3%, and freely excreted milt when removed from the net. An A. marmorata male also had enlarged testes with a GSI of 25.3% ( Fig. 1d ). These GSI values were also higher than values of artificially matured adults [26] ( ∼ 10–15%). The morphology of the testes of these naturally matured eels was comparable to the testes of artificially matured eels when examined under a light microscope. The testes contained a large amount of sperm, whereas cysts composed of spermatids and late type B spermatogonia were occasionally observed ( Supplementary Fig. S1f ), which was similar to histological observations of artificially matured testes with active spermiation. A unique characteristic of a crescent-shaped nucleus of eel sperm was also confirmed to be present in males collected in the spawning area, which was also reported to be present in artificially matured male eels [27] . Five of the collected male specimens excreted milt from the genital pore at collection, and histological observations showed that the spermatic duct of the testes was filled with sperm in all the males examined. The sperm motility of one A. japonica and one A. marmorata was confirmed onboard after capture, indicating that these eels were in spawning condition. No obvious difference in conditions of milt, such as viscosity, colour and morphology of spermatozoa, was observed between the males in the spawning area and artificially matured eels. These observations may suggest that the males in this study were fully matured and had participated in spawning during the new moon period when they were captured. The capture of spawning-condition eels also provided the first chance to examine some of their physiological parameters. Analyses of serum steroid hormone levels in A. japonica females collected on the night of the new moon (23 June 2009) found that 17α, 20β-dihydroxy-4-pregnen-3-one (DHP), thought to be an oocyte maturation/ovulation-inducing steroid hormone in this species [28] , was detected at considerable levels in the serum at about a 1 ng ml −1 concentration (range: 0.7–1.5, n =3), whereas DHP was not detected in artificially matured eels [29] . This concentration in wild adults is roughly equivalent to the level a few days after the DHP peaks that have been observed during the final maturation just before the ovulation and spawning of artificially mature adults [29] . Estradiol (female steroid hormone) was also detected at 2–3 ng ml −1 in the serum (range: 1.6–3.9, n =3), which was a level included in the range found in artificially matured eels at the mid- to late-vitellogenic stages [30] (range: 0.5–6.4, n =43). The level of 11-ketotestosterone (spermatogenesis-inducing steroid) was high (2–5 ng ml −1 ) in male eels caught in this study, similar to that in artificially matured males [27] . This type of information about the hormone dynamics of final maturation in wild eels will help to improve the egg and sperm quality of artificially matured eels and contribute to artificial glass eel production, which will facilitate conservation efforts for endangered eel species worldwide. Collections of eggs and hatched larvae The most unquestionable evidence of a spawning event by A. japonica near the West Mariana Ridge during the new moon was found in May 2009 when the first anguillid eel eggs of any species were found ( Fig. 4 ). Thirty-one eggs of A. japonica were collected in five tows at three stations in a grid of 25 stations centred around the first egg collection site ( Fig. 5 , Supplementary Fig. S2 ). The eggs were collected just south of the salinity front that was hypothesized to affect the latitude of spawning [2] , [31] , [32] , and in May 2009 the front crossed the seamount chain at around 13°N ( Fig. 5 ). The eggs that had been fertilized and were developing (termed 'embryos'; Fig. 4 ) were identified by morphology as possibly being A. japonica eggs because of their similarity with artificially fertilized eggs [33] , and were genetically confirmed to be A. japonica onboard the R/V Hakuho Maru within a few hours of the first egg collection using a real-time PCR system [34] that is designed to distinguish samples of Japanese eels from those of other similar species of eels onboard. 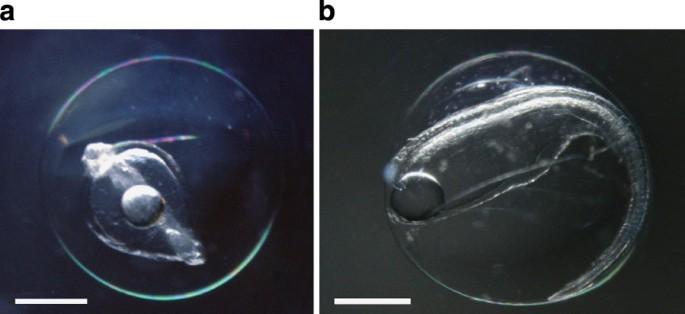Figure 4: Naturally spawned eggs of the Japanese eelAnguilla japonica. (a) Early-mid embryonic stage egg collected on 22 May 2009 near the West Mariana Ridge in the western North Pacific. (b) Late embryonic stage egg just before hatching collected on 23 May 2009 in the same area (Supplementary Fig. S2). Scale bars, 0.5 mm. Figure 4: Naturally spawned eggs of the Japanese eel Anguilla japonica . ( a ) Early-mid embryonic stage egg collected on 22 May 2009 near the West Mariana Ridge in the western North Pacific. ( b ) Late embryonic stage egg just before hatching collected on 23 May 2009 in the same area ( Supplementary Fig. S2 ). Scale bars, 0.5 mm. 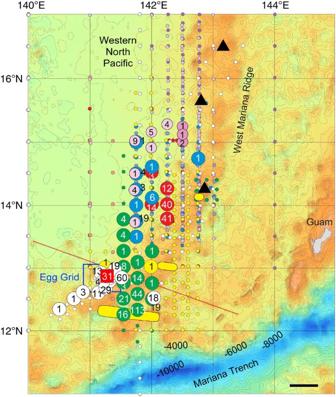Figure 5: Eel collection sites. Preleptocephalus catch locations of the Japanese eel,Anguilla japonica, in five different years (largest circles) and of the giant mottled eel,Anguilla marmorata, in 2 years (medium sized pink circles) are shown in relation to where adult eels were collected (three yellow ovals,Fig. 2), and the location of the grid of stations (blue rectangle) where 31A. japonicaeggs were collected (red square) just south of the salinity front (dotted red line) that crossed the southern end of the seamount chain in May 2009. The salinity front forms from higher tropical rainfall in the south, and its position appears to affect the latitude of spawning by adult eels2,31,32.A. japonicapreleptocephalus catches are shown for 2005 (ref.36; red circles), 2007 (blue circles), 2008 (green circles Leg 1, yellow circles Leg 2) and 2009 (KH-09-02, white circles) with large circles containing the number of preleptocephali collected, and small circles of the same colour showing no-catch stations during each of those cruises. Small circles of other colours were stations of other cruises in different months or years that did not collect preleptocephali (2005-Leg 4: orange, 2006-Leg 3: purple, 2006-Leg 5: light purple, 2007-Leg 3: light blue, 2009-KH-09-1: grey). Stations in which 29 preleptocephali ofA. marmorata, were collected in 2006 (darker pink) and 2007 (lighter pink) are also shown, and two otherA. marmoratapreleptocephali were collected at 13.5°N, 137°E in August 2006 (ref.15). Bathymetric depth is shown by colour, with shallower depths <4,000 m in yellow and brown and deeper depths in blue. Three shallow seamounts10are shown with black triangles. Black scale bar, 50 km. Full size image Figure 5: Eel collection sites. Preleptocephalus catch locations of the Japanese eel, Anguilla japonica , in five different years (largest circles) and of the giant mottled eel, Anguilla marmorata , in 2 years (medium sized pink circles) are shown in relation to where adult eels were collected (three yellow ovals, Fig. 2 ), and the location of the grid of stations (blue rectangle) where 31 A. japonica eggs were collected (red square) just south of the salinity front (dotted red line) that crossed the southern end of the seamount chain in May 2009. The salinity front forms from higher tropical rainfall in the south, and its position appears to affect the latitude of spawning by adult eels [2] , [31] , [32] . A. japonica preleptocephalus catches are shown for 2005 (ref. 36 ; red circles), 2007 (blue circles), 2008 (green circles Leg 1, yellow circles Leg 2) and 2009 (KH-09-02, white circles) with large circles containing the number of preleptocephali collected, and small circles of the same colour showing no-catch stations during each of those cruises. Small circles of other colours were stations of other cruises in different months or years that did not collect preleptocephali (2005-Leg 4: orange, 2006-Leg 3: purple, 2006-Leg 5: light purple, 2007-Leg 3: light blue, 2009-KH-09-1: grey). Stations in which 29 preleptocephali of A. marmorata , were collected in 2006 (darker pink) and 2007 (lighter pink) are also shown, and two other A. marmorata preleptocephali were collected at 13.5°N, 137°E in August 2006 (ref. 15 ). Bathymetric depth is shown by colour, with shallower depths <4,000 m in yellow and brown and deeper depths in blue. Three shallow seamounts [10] are shown with black triangles. Black scale bar, 50 km. Full size image Eggs were collected in a narrow time window ( Fig. 3b ) with similar developmental stages being obtained for two consecutive days (22–23 May). They were all at the embryonic stage, but ranged from early embryonic ( Fig. 4a ) to late embryonic stage just before hatching ( Fig. 4b ). They had egg yolk and one large oil droplet, and the egg capsule diameters were 1.49–1.71 mm (1.61±0.07 mm, mean±s.d.). These eggs were larger than those obtained from artificially spawned A. japonica females [33] (1.3–1.6 mm, IRAGO Institute, personal communication). On the basis of studies of artificially fertilized eggs that developed at different temperatures in the laboratory [33] , [35] and the temperatures just below the top of thermocline in the present study ( Fig. 6 ), the collected eggs were likely spawned on the night of 20–21 May, approximately 3.5 days before the new moon ( Fig. 3b ). 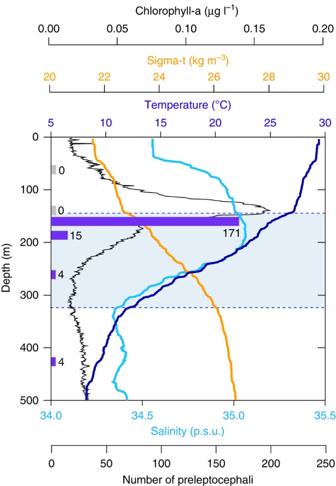Figure 6: Depth distribution ofAnguilla japonicapreleptocephali in relation to environmental conditions. The changes of each environmental parameter are plotted by depth from the ocean surface, and the number of preleptocephali that were collected at each depth stratum (65, 135, 163, 188, 265 and 425 m) is shown by purple bars (no catch tows are shown by zeros). The presence of the thermocline (shaded area between dotted lines) can be seen as the sudden change in water temperature (dark blue line) with depth. The large increase in chlorophyll concentration (black line) at around 150 m also occurred just above the top of the thermocline.Sigma-t(orange line) is a measure of water density that is calculated from both salinity (light blue line) and temperature. These data were collected on 23 May 2009 at the green circle inSupplementary Figure S2in the grid of 25 stations at the southern part of the West Mariana Ridge where the intensive survey for eel eggs and preleptocephali was made during 22–25 May 2009. Figure 6: Depth distribution of Anguilla japonica preleptocephali in relation to environmental conditions. The changes of each environmental parameter are plotted by depth from the ocean surface, and the number of preleptocephali that were collected at each depth stratum (65, 135, 163, 188, 265 and 425 m) is shown by purple bars (no catch tows are shown by zeros). The presence of the thermocline (shaded area between dotted lines) can be seen as the sudden change in water temperature (dark blue line) with depth. The large increase in chlorophyll concentration (black line) at around 150 m also occurred just above the top of the thermocline. Sigma-t (orange line) is a measure of water density that is calculated from both salinity (light blue line) and temperature. These data were collected on 23 May 2009 at the green circle in Supplementary Figure S2 in the grid of 25 stations at the southern part of the West Mariana Ridge where the intensive survey for eel eggs and preleptocephali was made during 22–25 May 2009. Full size image From 2005 (ref. 36 ) to 2009, ∼ 1,152 A. japonica preleptocephali were also collected near the seamount chain ( Supplementary Table S1 , Fig. 5 ). The timing of the collections ( Fig. 3c ) and otolith ageing data from daily increments (about 2–7 days after hatching) [36] indicated that spawning occured only during a 3-day period (2–4 days before the new moon) within the new moon period in each year. The catches occurred to the west of the Suruga Seamount in 2005 and 2007, and further south in 2008 and 2009 when the salinity front (dotted red line in Fig. 5 for May 2009) had moved southward, indicating that the spawning location varies among years and even months. There were also 29 A. marmorata preleptocephali collected in the northern part of this same area ( Fig. 5 ) during the new moon periods of July and August in 2006 and 2007 ( Supplementary Table S1 ), with 15 being collected at four of the same stations where A. japonica preleptocephali were collected in 2007 (ref. 15 ; Fig. 5 ). This species appears to have a wider seasonal range of spawning times than A. japonica , and two preleptocephali of A. marmorata were collected further west along 137°E in August 2006, indicating that this tropical anguillid may also sometimes spawn within a wider region [15] . Another interesting finding was that the mitochondrial DNA (mtDNA) control region sequences of 86 A. japonica preleptocephali collected in June 2005 included 77 different haplotypes, which showed that there were at least 77 females that had been spawning in the area where the preleptocephali were collected. This finding suggests that either many eels spawn in about the same area, such as in large aggregations, or that ocean currents and eddies can rapidly mix the eggs and larvae after spawning. Depth distribution of hatched larvae The presence of many preleptocephali within the egg grid sampled in May 2009 provided the opportunity to conduct horizontal tows targeting specific depth strata to evaluate their immediate post-hatching depth distribution, and thus determine the possible spawning depth of adult eels. Six replicate horizontal tows of a large midwater plankton trawl that fished at different depths on identical tracks showed a clear pattern of catches, with preleptocephali distributed in a vertically narrow depth stratum at ∼ 160 m and slightly deeper ( Fig. 6 ), whereas none were collected at 65 and 135 m. The 150-m depth layer was at the upper limit of the thermocline, and because recent laboratory research on the buoyancy of the eggs and preleptocephali of artificially spawned Japanese eels has indicated that these early life history stages are positively buoyant [13] , the eggs and larvae would have likely floated up to the top of the thermocline from slightly deeper depths. The concentrated vertical distribution of newly hatched larvae within a limited depth stratum ( Fig. 6 ) may suggest a limited range of upward movement of eggs during a short egg incubation time (38 h after fertilization at 23 °C) [33] after spawning, but the speed of upward movement of naturally spawned eggs is not known. The collection of large numbers of preleptocephali at 160 m provided the first clear evidence that spawning occurs below the top of the thermocline, and the capture of adult eels at depths between 160 and 300 m confirms this. Observations of the spawning behaviour of eels in the laboratory suggest that temperatures of 18–22 °C are optimal for successful spawning of A. japonica [11] , corresponding to depths of ∼ 200–260 m in Figure 6 . The survival rates of their larvae at different temperatures [35] also indicate that spawning is not much deeper than the layer just below the top of the thermocline (25–27 °C, Fig. 6 ), because artificially spawned newly hatched larvae showed the highest growth rate and lowest deformity rate at 25–28 °C (ref. 35 ). Many years after the sympatric spawning area of the Atlantic eels [37] was discovered [1] , this study provides the first detailed information about the reproductive biology of anguillid eels in the ocean. The catches of spawning-condition adults in the upper 300 m of the ocean, and the collections of eggs and recently hatched larvae at similar depths, indicate that the spawning depth of anguillid eels is probably within the warmer waters of the surface layer of the ocean. The observations of the morphological condition of spawning adults suggest that freshwater eels have the capacity for multiple spawning during a spawning season. However, their highly modified bodies and degenerated condition confirm that they have only one spawning season in their life and die after spawning a few times. The collections of adults, eggs and preleptocephali of A. japonica show a consistent pattern of spawning during the new moon nights of each month during their spawning season. The seamount chain and salinity front also seem to provide longitudinal and latitudinal cues for these eels to aggregate and spawn. Seamounts may have geomagnetic anomalies that provide landmarks for the migrating adults, because eels and other migratory animals are known to have a magnetic sense [38] , [39] that could be used to locate the spawning area [4] . The odour of deep-sea water upwelled by seamounts may also facilitate the aggregation of spawning adults using olfactory cues. The movable location of the salinity front [31] , [32] would then provide latitudinal cues for adults to cease their migration and search for breeding mates [2] . It appears that a remarkable set of oceanographic, geological and lunar cues are used by these eels to synchronize their spawning place and time at specific locations along the seamount chain each month during their spawning season. Synchronized spawning would enhance the fertilization rate, and spawning during the darkness of new moon nights would reduce the chances of predation on both adults and eggs. Also remarkable is that two anguillid species with significantly different adult body size, population structures [40] , [41] , [42] and freshwater habitat types in tropical and temperate regions have evolved migratory behaviours to use the same area for spawning [15] . Recent phylogenetic research has found that anguillid eels originated from deep-ocean midwater marine anguilliform species [43] , such as gulper eels, snipe eels and sawtooth eels, after which the ancestral anguillids invaded freshwaters for their juvenile growth period [23] . However, despite this remarkable change in the habitats used, anguillid eels still migrate back to their ancient spawning areas offshore [44] , while obtaining no additional nutrition during their long migrations [19] . These new findings about spawning-condition freshwater eels, the occurrence of their eggs and larvae, and their apparent spawning depths in this study can be combined with other valuable information obtained from tagging studies [6] , [7] , [8] , research using artificially matured adults and their larvae [11] , [12] , [13] , [14] , and from studies on the migratory abilities of these eels in the laboratory [45] , [46] . The information being gained from these new types of research can provide a better understanding of anguillid biology and life history, which can hopefully facilitate efforts to prevent further declines in the populations of these remarkable fishes that use both ocean and freshwater environments. Sampling for adult eels Sampling surveys for adult eels were conducted by the R/V Kaiyo Maru (Fisheries Agency) and the R/V Hokko Maru (Fisheries Research Agency) using large midwater trawl nets (Nichimo) along the southern part of the West Mariana Ridge ( Fig. 2 ) from May to August 2008 and May to June 2009 to learn about the reproductive ecology and spawning location of the Japanese eel and to facilitate conservation of this species. The maximum net mouth opening was 60 m in width and 50 m in height with a 7-mm mesh cod end for the Kaiyo Maru [3] , and 30 m in width and 30 m in height with a 17-mm mesh cod end for the Hokko Maru . A total of 62 horizontal-step tows were carried out mostly at night, while towing at 3–5 knots for 0.3–9.6 h during each deployment between depths of 132–766 m. Tows were carried out mainly at 160- to 300-m depths, where water temperature ranged from 13 to 23 °C. The duration of towing at each depth ranged from 0.3 to 3.0 h (mostly 1.5–2.0 h), which was monitored acoustically using a net sonde attached to the trawl. Genetic identification of adult eels The species identity of each adult eel caught in the spawning area was first determined onboard using morphological characters, and was genetically confirmed later in the laboratory using nucleotide sequence analysis of mitochondrial 16S rRNA genes (GenBank accession numbers AB445230 to AB445232, AB516443 and AB516444 for five specimens from 2008) using two primers ( Supplementary Table S2 ). Examination of adult eel characteristics Once eels were collected, they were photographed onboard the research vessels and biological parameters were measured, such as total length, head length, preanal length, predorsal length, body weight, eye diameter, pectoral fin length. The total lengths and body weights were compared between males and females of A. japonica using Mann–Whitney U -tests. After photographing and measuring the general biometrics, the adult eels were dissected onboard. The gonads of the eels were first examined and photographed. Whole gonad weight was measured to the nearest gram. GSI (percent relative gonad weight to body weight) was calculated. The condition factor [21] of each adult eel was calculated as body weight(g)/total length(cm) 3 ×1,000. Ovarian follicles were isolated with forceps and oocyte diameters were measured. Diameters of more than 100 randomly selected oocytes from each female eel were measured under a stereomicroscope using LEICA Image Manager (LEICA) and Image J (NIH) software. The diameters of ovulated eggs found in Eel No. 12 ( Table 1 ) were measured by the same method. Pieces of gonads and ovulated eggs were fixed in Bouin's solution for 1 day at 4 °C and stored in 70% ethanol onboard, and later in the laboratory they were embedded in paraffin, sectioned at 4 μm and stained with haematoxylin and eosin for histological observations. These sections were also used to measure the chorion thickness of oocytes. To ensure an accurate measurement, only oocytes with the nucleus exactly in the centre were used. The same procedure was used to measure the chorion thickness of oocytes of artificially matured eels held in the laboratory. A Mann–Whitney U -test was used to determine whether there were significant differences in chorion thickness between naturally and artificially matured eels. Pieces of gonad were also preserved in RNAlater solution and paraformaldehyde for future molecular and electron microscopic analysis, respectively. The oocyte developmental stages were assigned according to Yamamoto et al . [33] . Besides the gonads, we also preserved tissues such as pituitary, brain, liver, digestive tracts, swimbladder for future examination. Sagittal otoliths were also extracted for ageing and microchemistry studies, and the ages of the adult eels were determined later in the laboratory. The frontal section of the otoliths was ground and polished to the plane with the otolith core and the number of annual rings was counted under a polarized microscope [47] . The Sr and Ca concentrations in the otoliths of four A. japonica were measured in a line along the longest axis of each otolith from the centre to the edge using a wavelength-dispersive X-ray electron microprobe (JEOL, JXA-8900R) according to previous studies [48] . The mean Sr:Ca ratios were then calculated for each otolith and the general type of habitat used by each eel could be estimated as being freshwater, estuarine or marine habitats [48] . Measurement of eel hormones Hormone levels in the blood of the spawning-condition male and female A. japonica were measured. Immediately after they were removed from the trawl and brought into the laboratory onboard the research vessel, a syringe was used to obtain blood samples from the caudal vasculature of each eel. Serum was separated by centrifugation at 2,000 g for 5 min and then stored at −80 °C until analysis. In the laboratory back on land, the levels of DHP and estradiol in the females, and 11-ketotestosterone in males, were measured by time-resolved fluoroimmunoassays, as described elsewhere [49] . Sampling for eggs and leptocephali Sampling for the larvae of the Japanese eel has occurred historically in many regions of the western North Pacific [2] , [36] , [50] , [51] , but recent efforts have mostly been just west of the West Mariana Ridge. Since 2005, sampling was conducted with single oblique tows (0–300 m deep) of the large ORI-BF (Ocean Research Institute, Big Fish) ring net (3 m in diameter) with 0.5-mm mesh, deployed from the R/V Hakuho Maru (JAMSTEC, Atmosphere and Ocean Research Institute). In 2005, 178 stations were sampled and preleptocephali were collected at five stations ( Fig. 5 , Supplementary Table S1 ) to the west of the Suruga Seamount [36] . In 2007, out of 167 stations, preleptocephali were caught at nine stations, and, in 2008, they were caught at 16 out of 308 stations (14 in Leg 1, 2 in Leg 2). In 2009, the primary effort to collect Japanese eel eggs and larvae using the large ring net was made during two Hakuho Maru cruises in April and May. In the first cruise KH-09-1, 90 stations were sampled from 18 to 30 April 2009, but no eggs or preleptocephali were collected. During the second cruise KH-09-2, 86 stations were sampled near the seamount chain from 17 to 27 May 2009 and eggs were collected for the first time on 22 May during sampling along the ridge (12.5°N–16.5°N), which was followed by collections of many preleptocephali from the same spawning event. An intensive survey was then conducted in a grid of 25 stations and in other nearby areas, with 753 preleptocephali being collected at 27 stations in KH-09-2 ( Fig. 5 , Supplementary Fig. S2 ). Additional sampling was then conducted further west along 137°E until 31 May, but no additional eggs or preleptocephali were collected. After each tow of the net, leptocephali or eggs were sorted fresh out of the plankton samples and examined morphologically. Larger leptocephali were morphologically identified by counting the number of their myomeres (muscle segments), whereas some eggs and small preleptocephali were genetically identified onboard [34] . In 2009, eggs were photographed using a Nikon SMZ1500 dissecting microscope and a Nikon DMX1200F digital imaging system (Nikon). Specimens were either preserved in 99% ethanol or were frozen to enable later DNA or otolith analyses. Depth distribution of preleptocephali To evaluate the depth distribution of newly hatched preleptocephali, six tows at six different depth layers were carried out on 23 May 2009 (10:34–17:32) at the same location within the tight grid of stations around the egg catch area ( Supplementary Fig. S2 ). The ORI-BF net was deployed to the target depth and towed horizontally at that depth for 20 min and then retrieved to the surface. As the net was open while moving to and from the target fishing depth, some contamination from shallower depth layers was possible; however, in this case, no larvae were collected in the two tows in the upper 135 m, which established that the larvae were distributed deeper than 135 m ( Fig. 6 ). Hydrographic profiles Conductivity, temperature and depth (CTD) hydrographic profiles were obtained using a CTD system (Sea-Bird Electronics, USA) during each cruise. In May 2009, the Tenyou Maru (National Fisheries University) made a transect of CTD stations east of the seamount chain along 143.5°E. The position of the salinity front was distinguished by the location of 34.5 p.s.u. salinity at the sea surface [31] , [32] in this transect (12.5°N) and in a Hakuho Maru transect along 140°E (13.5°N; Fig. 5 ). The salinity front was used as a reference to determine the likely area for intensive larval sampling by Hakuho Maru just before the new moon when the salinity front crossed the seamount chain. CTD profiles were also obtained at the station where the larval depth distribution study was conducted. In addition, within the tight grid of stations where eggs were collected, six X-CTD (expendable CTD probes, Tsurumi Seiki) were deployed to obtain additional hydrographic data. Onboard genetic identification of eggs and larvae To determine whether Japanese eel preleptocephali or eggs were collected, some specimens were tested onboard Hakuho Maru using a real-time PCR A. japonica sequence detection system established for this species [34] . In May 2009, real-time PCR was conducted on the first 2 eggs that were collected, before deciding to conduct intensive sampling in a grid around the original catch location. Briefly, the methods of this type of analysis are that DNA was extracted from each egg or larva and used for PCR with an A. japonica -specific primer pair and a fluorescent-labelled oligo probe [34] ( Supplementary Table S2 ). The reactions were carried out in a real-time-monitoring thermal cycler (ABI 7300 Real-Time PCR System), and amplification was quantified at each reaction cycle. A positive ( A. japonica ) or negative (another species) result of the PCR was determined according to whether the amplification efficiency reached the expected level [34] . However, the results were confirmed later in the laboratory on land by determining the DNA nucleotide sequences of the 16S rRNA gene of mtDNA. All of the remaining 28 eggs and most of the preleptocephali from each year were confirmed to be A. japonica using their DNA sequences. Genotype analysis of preleptocephali The mtDNA control region of 86 preleptocephali collected in June 2005 was examined to determine their parentage history. This analysis found 77 different haplotypes [40] that had 1–16 site differences among 511 base pairs of aligned mtDNA sequences. The total DNA samples were extracted from preleptocephali, and used for PCR to amplify a part of the control region with the PCR primers L15774 (ref. 52 ) and H16498 (ref. 53 ; Supplementary Table S2 ). The sequencing reactions were carried out with the same primers as those used for PCR. All sequences were automatically aligned using Clustal X [54] and manually compared using DNASIS ver. 3.7 (Hitachi Software Engineering). Accession codes: Mitochondrial 16S rRNA sequences have been deposited in the GenBank Nucleotide Core Database under the accession numbers AB445230 , AB445231 , AB445232 , AB516443 and AB516444 . How to cite this article: Tsukamoto, K. et al . Oceanic spawning ecology of freshwater eels in the western North Pacific. Nat. Commun. 2:179 doi: 10.1038/ncomms1174 (2011).